Arctic tree rings as recorders of variations in light availability Annual growth ring variations in Arctic trees are often used to reconstruct surface temperature. In general, however, the growth of Arctic vegetation is limited both by temperature and light availability, suggesting that variations in atmospheric transmissivity may also influence tree-ring characteristics. Here we show that Arctic tree-ring density is sensitive to changes in light availability across two distinct phenomena: explosive volcanic eruptions ( P <0.01) and the recent epoch of global dimming ( P <0.01). In each case, the greatest response is found in the most light-limited regions of the Arctic. Essentially no late 20th century decline in tree-ring density relative to temperature is seen in the least light-limited regions of the Arctic. Consistent results follow from analysis of tree-ring width and from individually analysing each of seven tree species. Light availability thus appears an important control, opening the possibility for using tree rings to reconstruct historical changes in surface light intensity. Records derived from tree rings figure prominently among reconstructions of surface temperature because they are well distributed on land, have annual resolution and extend back centuries or even millennia [1] . In Arctic regions, the maximum density of wood formed in the late-growing season has a particularly strong relationship with temperature, tending to be denser during warmer years [2] , [3] , [4] . The isotopic composition of wood is known to be influenced by light availability [5] , and here we explore the hypothesis of a broader imprint of light variability on wood formation [5] , [6] . Standard physiological models describe photosynthesis as being increasingly sensitive to variations in light availability in low-light environments [7] , [8] , and light addition experiments in tropical forests have shown increased growth in response to above-canopy light addition on cloudy days [9] . No such direct experimental data are available in the Arctic, but it is possible to examine growth responses to natural variations in light availability. Decreases in the magnitude of light reaching the Arctic surface are observed as a result of several processes. First, explosive volcanic eruptions loft SO 2 into the upper atmosphere where it reacts to form aerosols that decrease the intensity of sunlight reaching Earth’s surface. Low-latitude eruptions generally cause the greatest dimming of Arctic radiation 2 years after the eruption because of slow poleward migration in the stratosphere [10] . Second, anthropogenic aerosol emissions increase the scattering and absorption of sunlight. Finally, changes in clouds—possibly related to aerosols acting as cloud condensation nuclei—also alter the scattering and absorption of sunlight. Some combination of changes in aerosols and clouds decreased surface intensity during the second half of the 20th century [11] , [12] , [13] . The magnitude and timing of this dimming vary across the globe, with the greatest Arctic dimming estimated to have occurred between 1955 and 1975 with a total reduction in the range of 10% (refs 12 , 14 ) ( Supplementary Fig. 1 ), about half the Arctic dimming estimated to have followed the Mount Pinatubo eruption [12] , [14] . Following [4] and [15] , we analyse the Schweingruber collection of tree-ring maximum latewood density chronologies [16] over the area north of 50°N (hereafter the Arctic). Tree-ring densities are focussed on because they respond more exclusively to climate anomalies during the year of growth [17] and have a stronger correlation with local variations in daily average temperature [15] . We find that the spatial pattern of the tree-ring response to volcanism and to global dimming is consistent with the hypothesis that tree-ring properties are sensitive to changes in light availability. Classification of chronologies by limitation regime Density records are normalized (see Methods) and grouped into four categories according to an estimate of the degree to which temperature and light availability limits growth [18] . Specifically, records are categorized as having relatively high- or low-light limitation, which follows from climatological cloud cover, depending on whether the corresponding location falls above or below the sample median Arctic value. A similar division is made according to high- or low-temperature limitation ( Fig. 1 ). For simplicity, these sectors will be referred to as cloudy or clear, and cold or warm. Although water limitation on growth has been identified in parts of Alaska [17] , it appears generally less of a constraint on Arctic growth than temperature or light [18] . 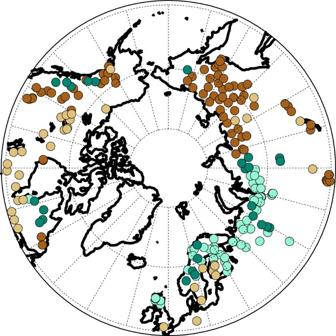Figure 1: Grouping of Arctic tree-ring density chronologies by strength of light and temperature limitation. Each circle represents one of the tree-ring chronologies used in this study. Chronologies are distinguished according to being from sectors that are cloudy and cool (dark green), cloudy and warm (light green), clear and cool (dark brown), and clear and warm (light brown). Figure 1: Grouping of Arctic tree-ring density chronologies by strength of light and temperature limitation. Each circle represents one of the tree-ring chronologies used in this study. Chronologies are distinguished according to being from sectors that are cloudy and cool (dark green), cloudy and warm (light green), clear and cool (dark brown), and clear and warm (light brown). Full size image Explosive volcanism To examine the effects of volcanic eruptions on tree-ring density, we extract 13-year segments from each density record centred on the 15 biggest volcanic eruptions identified in ice cores from 1300–1950 (ref. 19) [19] . Averaging over all such segments in each of the four sectors shows a general decrease in tree-ring density following volcanic eruptions ( Fig. 2a ) but with a significantly greater response in the cloudy than clear sectors ( P <0.01, using a t -test and accounting for spatial covariance, see Methods). The cloudy-cold sector shows the largest decrease, consistent with low-temperature and low-light environments being more sensitive to further reductions in both quantities. Furthermore, the cloudy-warm sector shows a greater response than the clear-cold one, suggesting that light limitation may be the more important of the two influences in the Arctic, at least with respect to volcanism. 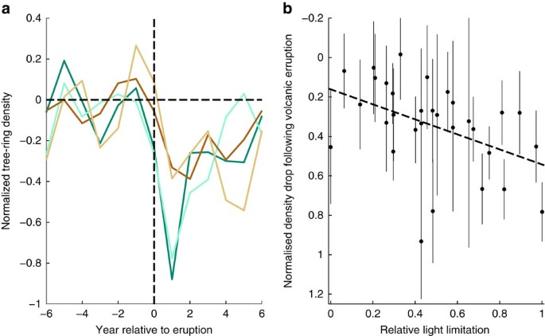Figure 2: Tree-ring density response to volcanism. (a) Tree-ring density anomalies across large volcanic eruptions averaged according to the four sectors given inFig. 1. Averages comprise all complete tree-ring density segments centred on the 15 largest volcanic eruptions between 1300–1950 (ref. 19)19. Cloudy regions of the Arctic (dark green and light green) show a greater negative anomaly than the clear regions (dark brown and light brown). Values are anomalies relative to mean density in the 5 years preceding a volcanic eruption. (b) Volcanic density drop versus local light limitation averaged over the 15° × 15°-grid boxes indicated inFig. 1. Density drop following a volcanic eruption is measured as the tree-ring density in the 5 years before an eruption minus the 2 years after a volcanic eruption, and the trend line is a least-squares linear fit. Vertical bars indicate the 95% confidence interval. Figure 2: Tree-ring density response to volcanism. ( a ) Tree-ring density anomalies across large volcanic eruptions averaged according to the four sectors given in Fig. 1 . Averages comprise all complete tree-ring density segments centred on the 15 largest volcanic eruptions between 1300–1950 (ref. 19) [19] . Cloudy regions of the Arctic (dark green and light green) show a greater negative anomaly than the clear regions (dark brown and light brown). Values are anomalies relative to mean density in the 5 years preceding a volcanic eruption. ( b ) Volcanic density drop versus local light limitation averaged over the 15° × 15°-grid boxes indicated in Fig. 1 . Density drop following a volcanic eruption is measured as the tree-ring density in the 5 years before an eruption minus the 2 years after a volcanic eruption, and the trend line is a least-squares linear fit. Vertical bars indicate the 95% confidence interval. Full size image It is also useful to compare light limitation and the tree-ring density response with volcanism as a function of space. We again find a significant relationship between the strength of local light limitation and the density decrease following a volcanic eruption (Pearson’s R =0.31, P <0.01, one-sided), with a greater response occurring in the cloudiest locations, as expected [7] , [8] . The sense of the relationship also becomes more pronounced once records are more evenly weighted across space through averaging within 15° × 15° grid boxes ( Fig. 2b ). This size generally ensures more than one record within each box and gives largely independent realizations because seasonal temperature anomalies have an ~1,000 km covariance length scale (see Methods). After averaging, the correlation between light limitation and the density response increases to R =0.44 ( P <0.01, one-sided). Note that the consistent P -values across the binned and unbinned results is expected as a consequence of exchanging numbers of samples for less noisy averages. There are two outliers in the light availability analysis along the eastern edge of the Hudson Bay, possibly arising from noise in the records. Regional variability in radiation and temperature is also expected, however, because volcanic eruptions can change atmospheric circulation patterns, with consequent changes in cloud cover [10] . Period of divergence A similar test for the influence of light limitation on ring density is possible over the period of Arctic dimming. Importantly, during this period we can isolate variations in tree-ring density that diverge from temperature because of the availability of instrumental temperature records. Synthetic experiments indicate a more powerful test for light limitation is possible when using linear regression to remove the temperature component, as opposed to a differencing approach more commonly used for diagnosing divergence [15] , [20] (see Methods). Accordingly, we regress out temperature and then use the negative trend in residual tree-ring density during the 1955–1975 period as a metric to test for a light response. The 1955–1975 temperature trend averaged over the location of our tree-ring records is positive (0.13 °C per decade), as compared with an average tree-ring density trend that is negative (−0.21 standard deviations per decade). This period coincides with when the strongest decrease in light availability occurs in the Arctic [12] , [14] ( Supplementary Fig. 1 ) and when ref. 15 reports divergence between temperature and Arctic tree-ring records. The regression method both partitions variance between signal and noise differently than the more common method and gives a different spatial pattern than reported in ref. 15 , with the strongest trends in residual density centred on the Polar Ural mountains. Trends in residual tree-ring density are more negative in the cloudy Arctic sectors than the clear ones ( Fig. 3a ). A test of the trends in residuals against a null hypothesis of a distribution about a mean of zero indicates highly significant negative trends in the two cloudy sectors ( P <0.01), significant negative trends in the clear-warm sector ( P =0.03), and no trend in the clear-cold sector. There is also a significant correlation between the magnitude of the trend in residuals and light limitation ( R =0.32, P <0.01) that increases after averaging within the 15° × 15°-grid boxes ( R =0.65, P <0.01, Fig. 3b ). The largest response occurs in the cloudiest regions and reaches magnitudes similar to those associated with the response to volcanism ( Figs 2 , 3 ). In contrast, no response to dimming is detected in the most cloud-free Arctic regions, where light limitation is weakest. The absence of a response in the least cloudy regions is also consistent with the absence of divergence in subarctic regions where there is even greater light availability [21] , [22] . 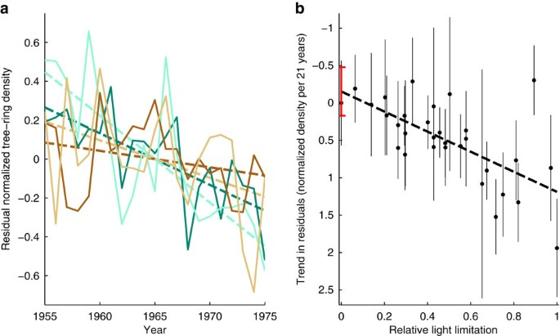Figure 3: Tree-ring residual density trends during Arctic dimming. (a) Tree-ring density averaged within each of the four sectors given inFig. 1after removing the component linearly related to local temperature. Trends are from a least-squares linear fit and are most negative in the cloudy regions (dark green and light green) and least in the clear ones (dark brown and light brown). (b) Light limitation versus trend in residual density (defined here as the negative trend in residual density) averaged over 15° × 15° grid boxes (black dots). None of the five negative values are significantly different from zero, as indicated by their 95% confidence intervals (vertical bars). The major outlier in the upper-right quadrant is from a Scottish collection of tree-ring chronologies. The dashed black line is from a least-squares linear fit. Note that the 95% confidence interval for they-intercept (red line) encompasses zero, indicating that the clearest Arctic regions show no trend in residual density over the dimming period. Vertical bars indicate 95% confidence uncertainty range. Figure 3: Tree-ring residual density trends during Arctic dimming. ( a ) Tree-ring density averaged within each of the four sectors given in Fig. 1 after removing the component linearly related to local temperature. Trends are from a least-squares linear fit and are most negative in the cloudy regions (dark green and light green) and least in the clear ones (dark brown and light brown). ( b ) Light limitation versus trend in residual density (defined here as the negative trend in residual density) averaged over 15° × 15° grid boxes (black dots). None of the five negative values are significantly different from zero, as indicated by their 95% confidence intervals (vertical bars). The major outlier in the upper-right quadrant is from a Scottish collection of tree-ring chronologies. The dashed black line is from a least-squares linear fit. Note that the 95% confidence interval for the y -intercept (red line) encompasses zero, indicating that the clearest Arctic regions show no trend in residual density over the dimming period. Vertical bars indicate 95% confidence uncertainty range. Full size image Robustness It appears unlikely that the relationship between light availability and variations in tree-ring density stem from age-growth artifacts. The spatial pattern associated with the trends in residual density is strongly correlated with the magnitude of the volcanic response ( R =0.66, P <0.01, see Supplementary Fig. 2 ), and volcanic responses are little influenced by age-growth artifacts because they are brief and distributed throughout the record. Furthermore, qualitatively identical results are obtained if the signal-free detrending approach [23] is first applied to our collection of records ( Supplementary Fig. 3 ). Elsewhere it has been suggested that tree-ring records from marginal thermal environments generally underestimate the influence of volcanic events [24] , [25] . We have proposed a rather different scenario—that tree-ring records from marginal light environments show a relatively greater response to volcanic events because of sensitivity to both temperature and a decrease in light availability that is not entirely compensated for by an increased fraction of diffuse light. Although our and ref. 24 models of tree-ring response need not contradict one another, there is the possibility that covariance between light and temperature environments would lead to incorrect attribution if not otherwise accounted for. We have thus recalculated our volcanic response estimates as a function of light limitation excluding the two cold regions in order to minimize potential covariance between the proposed mechanisms. We find no reduction in the correlation between gridded light limitation and the tree-ring density response to volcanic eruptions ( R =0.45, P <0.03, one-sided). Similar results hold when we exclude the 50% of chronologies with coldest peak monthly summer temperature ( R =0.52, P <0.01, one-sided), which are predicted to have the greatest response by ref. 24 . Our results are robust to removing portions of the data because sensitivity to volcanism grades continuously with light limitation throughout the dataset. Although it is beyond the scope of our present study to evaluate the merits ref. 24's proposed mechanism, these additional test results indicate that such an effect does not compromise our results. These additional tests are also consistent with the close correspondence that we find between volcanic and dimming-era responses, where the latter would be less susceptible to ref. 24's hypothesized model. It has also been noted that divergence between temperature and tree-ring density is found more prevalently in shade-tolerant species of trees [26] , consistent with a greater response to dimming occurring in light-limited regions, but raising the question of whether physiological differences between species influence the response. Breaking the analysis down according to the seven different species that are abundantly present shows a response to dimming within each species that is consistent with our general finding of environmental light limitation modulating the strength of the response to perturbations in light availability. Correlations between divergence and light availability are positive and highly significant ( P <0.01) for three species, and positive and significant ( P <0.02) for one other. The remaining three species also show a positive correlation but not a statistically significant one, possibly because these span a relatively small range of light limitation values ( Fig. 4 ). In all cases, the relationship between light limitation and the response to dimming for individual species is consistent with no response in the clearest regions of the Arctic. 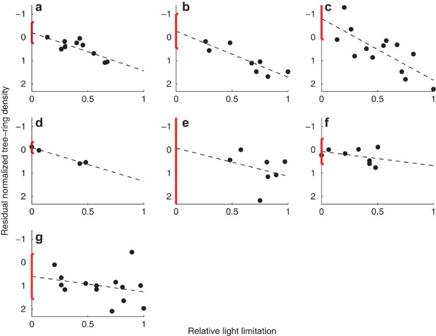Figure 4: Tree-ring residual density trends by species. Light limitation versus trend in residual density (defined here as the negative trend in residual density) averaged over 15° × 15° grid boxes, but with analysis done separately for each of the seven species represented within the data collection that have members present in at least three grid boxes. All species show a positive correlation between normalized light limitation and divergence. This correlation is highly significant for (a) Larix gmelinii (R=0.77,P<0.01), (b) Larix sibirica (R=0.87,P<0.01) and (c) Picea obovata (R=0.76,P<0.01). (d) Picea mariana has a strong correlation but lower significance (R=0.99,P<0.02) because of the small number of datapoints (N=4). The relationship is positive, but not significant at theP=0.05 level for (e) Picea abies, (f) Picea glauca and (g) Pinus sylvestris. The 95% confidence interval for they-intercept (red line) encompasses zero in all cases. Figure 4: Tree-ring residual density trends by species. Light limitation versus trend in residual density (defined here as the negative trend in residual density) averaged over 15° × 15° grid boxes, but with analysis done separately for each of the seven species represented within the data collection that have members present in at least three grid boxes. All species show a positive correlation between normalized light limitation and divergence. This correlation is highly significant for ( a ) Larix gmelinii ( R =0.77, P <0.01), ( b ) Larix sibirica ( R =0.87, P <0.01) and ( c ) Picea obovata ( R =0.76, P <0.01). ( d ) Picea mariana has a strong correlation but lower significance ( R =0.99, P <0.02) because of the small number of datapoints ( N =4). The relationship is positive, but not significant at the P =0.05 level for ( e ) Picea abies, ( f ) Picea glauca and ( g ) Pinus sylvestris. The 95% confidence interval for the y -intercept (red line) encompasses zero in all cases. Full size image Divergence has also been diagnosed in records of Arctic tree-ring width [15] , and we have repeated our analysis using the width chronologies available in the Schweingruber collection of tree-ring data [16] . Consistent with the foregoing results, light limitation is significantly and positively correlated both with the pattern of decreasing widths following volcanic eruptions ( R =0.49, P <0.01) and the pattern of trends in residuals during the period of modern Arctic dimming ( R =0.34, P <0.04, Supplementary Fig. 4 ). Mechanistic framework The parallel results that we find for tree-ring width and density suggest a simple interpretation of our basic result that light variations influence tree rings that can be described in terms of the Vaganov–Shashkin tree-ring model [3] . In this model, growth rate in temperature-limited regions is proportional to the product of a temperature-limitation factor and a measure of local incoming solar radiation. Solar radiation can be interpreted to control growth through enabling photosynthesis or influencing growth through signalling the timing and duration of growth stages. Application of the Vaganov–Shashkin model to central Siberian taiga trees [3] , for example, led to the inference that initiation of growth is largely controlled by temperature while the cessation of growth is controlled by light, which also provides a mechanism for how temperature and light may together influence the rate and duration of cambial activity and lignification. We also find that sensitivity to variations in radiation are stronger in environments having greater light limitation, a feature not included in the Vaganov–Shashkin tree-ring model, but which may help to explain variations in whether divergence is expressed across different studies. This also suggests that trees sampled at the periphery of stands with good light exposure may suffer less from dimming than those in more enclosed interior locations, and such careful site selection may explain why recent tree-ring studies [20] , [27] , [28] have a noted consistency with temperature. A further consideration is the partition of light into direct and diffuse components. Diffuse light may drive greater photosynthesis through penetrating more evenly into the canopy [29] . Volcanic aerosols and clouds are expected to increase the fraction of diffuse solar radiation reaching the surface, but our results indicate that the greater efficiency associated with diffuse light incompletely compensates for overall light loss, especially in the cloudy section of the Arctic. The cloudy sections receive, on average, 59% of their light as diffuse and may benefit less from additional scattering than the clear sections, which receives 48% of their light as diffuse (see Methods). Such a dependent response would be consistent with findings that a forest in an even less-diffuse environment at mid-latitudes experienced greater growth on cloudless days after the 1991 Mount Pinatubo eruption [30] . Note, however, that the influence of industrial aerosol changes during the period of divergence is more uncertain because aerosols are estimated to have become more absorbing during this interval [31] . There are several more general implications of these findings. First, geoengineering proposals to intentionally inject aerosols into the stratosphere to cool the planet [32] may have the unintended side-effect of decreasing tree growth and carbon uptake in already light-limited regions. Second, whenever surface light availability and temperature diverge, we should also expect divergence between temperature and reconstructions of that temperature when using tree-ring records that are light limited. A recent multi-proxy study of Arctic climate found no evidence for divergence in the 600 years before 1950 (ref. 33) [33] , but it cannot be excluded that undetected divergence is present or that divergence occurred at earlier times. Further analysis incorporating indications of changes in light availability using stable carbon isotopes [5] , [34] , [35] , [36] , [37] , [38] , [39] or the covariance between light and moisture in water-limited trees [40] would be useful. Finally, sensitivity to light variations complicates the interpretation of tree-ring chronologies but also suggests that tree-ring density and width records from low-light environments may aid in the reconstruction of past changes in surface radiation. Instrumental temperature Temperature variability at the location of each tree-ring chronology is estimated through optimally interpolating [41] monthly average temperature anomalies from the Climate Research Unit’s gridded land temperatures [42] to the location of each chronology using a temperature decorrelation length scale of 1,000 km (ref. 43 ). Gridded temperatures are assumed to reside at the centre of the grid box. April–September averages are used, in accord with the seasonal average that ref. 44 found to be optimal. Tree-ring density Tree-ring data are from the Schweingruber collection [16] , where we analyse data that are north of 50°N and that cover at least 70 years in the interval up to and including 1975, after which data coverage falls off precipitously. Each tree-ring chronology is normalized to unit variance over the pre-1950 epoch to avoid introducing artifacts associated with the period of dimming, though our results are qualitatively unchanged if we instead normalize over the entire record or normalize after masking out years that are especially influenced by volcanic eruptions. Nor does application of the generalized exponential (that is, Hugershoff) method used by ref. 15 or the signal-free method of ref. 23 have consequence for our findings, indicating that results are independent of age-growth effects ( Supplementary Fig. 3 ). Similar results follow from analysis of tree-ring width ( Supplementary Fig. 4 ) and mean latewood density ( Supplementary Fig. 5 ). Light and temperature-limitation estimates Gridded values of relative light and temperature limitation on photosynthesis are taken from ref. 18 , which reports global values at half-degree resolution. Because light and temperature-limitation values are provided at higher resolution and are more spatially complete than the temperature data, a nearest neighbour approach is used in relating each tree-ring density record to light- and temperature-limitation values. The collection of light- and temperature-limitation values associated with tree-ring density records are rescaled to values between 0 and 1 over the collection of 15° × 15° gridded chronologies. Rescaling does not distort the metric because the initially reported values are also unitless indices. Gridded temperature and light limitations are estimated in ref. 18 from climatological temperature and cloud cover. Light limitation is estimated as linearly proportional to cloud cover above a minimum threshold of 10%, and temperature limitation is estimated as linearly proportional to minimum temperature rescaled to zero below −5 °C, linearly increasing from −5 °C to +5 °C, and equal to one above 5 °C. Diffuse and direct radiation The climatological fraction of surface solar insolation that is diffuse is estimated as the ratio of diffuse to total surface insolation across the available Global Energy Balance Archive stations in the Arctic [45] . There are 100 Arctic stations for which both diffuse and total insolation are reported and which meet the provided quality-control checks. April–September average values are considered in accord with the hypothesis that growing season insolation influences tree-ring density and for parity with the seasonal average used for temperature data [44] . Records vary in length from 1–45 years, and omitting those stations with only 1 or 2 years of record length has essentially no influence on results. Light limitation at each location where insolation is observed is estimated as the value at the nearest gridded value reported by ref. 18 . As expected, the diffuse fraction generally increases in more light-limited locations ( Supplementary Fig. 6 ). Testing the volcanic response The tree-ring width or density response to volcanism for each chronology is calculated as the average decrease in tree-ring width or density during the year of eruption and the following year, relative to the average for the 5 years preceding the volcanic eruption. The response to volcanism in each 15° × 15°-grid box is estimated as the weighted average of the volcanic response of each chronology in the grid box, where each chronology is weighted in proportion to the number of eruptions it samples. Uncertainty for each chronology is calculated as the standard error of the mean volcanic response across all eruptions with chronologies sampling fewer than two eruptions excluded. All correlations cited in the main text of the manuscript are Pearson’s R coefficients. Spearman’s rank correlation was also used for the volcanic tests on account of questions regarding whether these are influenced by non-normality and was found to give consistently significant correlations between the volcanic density drop and local light limitation for both point estimates ( ρ =0.3, P <0.01) and 15° × 15° gridded estimates ( ρ =0.47, P <0.01). The median chronology samples 7 of the 15 volcanic eruptions used in this study. To assess the influence of the differential temporal coverage of chronologies, we repeat the analysis using a reduced ‘fixed eruptions network’ of 107 chronologies that all sample an identical collection of eight major volcanic events, and we obtain consistent results ( Supplementary Fig. 7 ). Effective spatial degrees of freedom As recommended [46] , we estimate effective spatial degrees of freedom (ESDOF) using moment matching when comparing realizations of a mean value, using eigenvalues when assessing correlations, and using the harmonic mean of these two estimates when comparing realizations. The ESDOF is the number of independently varying spatial patterns in a time-varying field [46] . The degrees of freedom of a given test is ESDOF− k , where k is the number of parameters calculated as intermediate steps in estimating the test statistic. P -values for ungridded correlations are estimated using a t distribution with degrees of freedom determined as the ESDOF −2, where and with the ESDOF estimated using the eigenvalue approach [46] . P -values for Spearman’s rank correlation coefficients ( ρ ) are estimated in the same manner with . P -values for residual trends over the period of dimming are estimated from the distribution of residual trends found within each sector with ESDOF estimated separately within each sector using the harmonic mean method [46] . P -values for differences between the volcanic response in the clear and cloudy sectors are estimated using a paired sample t -test with N -1 degrees of freedom, where N is the number of volcanic eruptions considered. ESDOF are estimated separately for tree-ring density and the residual tree-ring density after linearly regressing out temperature, and are calculated separately within each sector where appropriate. For tree-ring density, we estimate 79, 94 and 86 ESDOF for the moment matching, eigenvalue formula and harmonic mean methods, respectively. For residual density variability, we respectively estimate 35, 56 and 43 ESDOF. ESDOF for individual quadrants are given in Supplementary Table 1 . Spatial aggregation Averaging within 15° × 15° grid boxes gives largely independent realizations because temperature anomalies have a spatial covariance of ~1,000 km on seasonal time scales [43] . All aggregation methods that we considered, however, give similar results. For example, binning into an equal number of bins as used in the spatial analysis, but instead by the magnitude of light limitation, which is more optimal from a noise reduction perspective, results in even stronger correlations between light-limitation strength and both volcanic response ( R =0.82, P <0.01) and trends in residual density over the period of dimming ( R =0.69, P <0.01). Water limitation Although water limitation is generally weak in the Arctic, covariation between tree-ring growth and precipitation has been noted at a handful of Arctic locations, primarily in Alaska [17] . These correspond to the regions of the Arctic where photosynthesis is estimated to be most limited by water availability [18] . We detect no large-scale correspondence, however, between water limitation and either the volcanic response ( R =−0.25, P =0.19, two-sided) or the negative trend in residual density over the dimming period ( R =−0.14, P =0.45, two-sided), consistent with the expectation that water limitation is not widespread in the Arctic [18] . A two-sided test is used because the sign of water-stress change may vary given potentially competing changes in precipitation and evaporation. Factoring out temperature Identification of divergence between temperature and tree-ring records was accomplished through a scaling and differencing approach in previous studies [15] . Our experiments with synthetic records (described below), however, indicate that a regression-based approach for removing the temperature component is superior. In particular, these synthetic experiments indicate that regressing out temperature variability is almost twice as likely to lead to detecting the presence of a light-limitation influence on tree-ring records, if such an influence is truly present. We, therefore, use linear regression to remove the component of temperature associated with each tree-ring density or width record such that residuals are uncorrelated with temperature. Comparison with method of Briffa et al The statistical power of a test to identify a spatial pattern associated with global dimming [11] , [12] , [13] , [14] , [31] , [45] , [47] , [48] , [49] , [50] depends on the details of how records are normalized and how the response is measured. Methods developed for reconstructing temperature variability from tree rings, for instance, are not necessarily optimal for identifying the spatial pattern associated with a second non-noise process. This distinction prompts an in-depth examination of different methods. Briffa et al. [15] estimate a spatial pattern of residuals, which they refer to as ‘divergence’ through a series of normalization and differences. Specifically, each tree-ring density chronology is normalized to zero mean and unit variance over the 1901–1940 period. Chronologies are then averaged regionally, and means and variance are renormalized with respect to the 1881–1940 period. Similarly, temperature records are regionally averaged and then normalized to zero mean and unit variance between the 1881–1940 period. A correction is also applied to the variance of both the tree-ring density and temperature records according to their effective degrees of freedom. The normalized regional temperature is then subtracted from the normalized regional density chronology to yield a difference time series. Divergence is calculated from this difference time series as the 1975–1985 average minus the 1935–1945 average. In this study, the response to dimming is estimated by normalizing all density chronologies to zero mean and unit variance using all values before 1950. Each normalized chronology is then linearly regressed against local temperature over the full length of overlap between the thermometer and tree-ring record, usually encompassing a period between approximately 1850–1975. After removing the temperature component, the least-squares best-fit linear trend between 1955–1975 in the residual tree-ring density record is calculated. The interval 1955–1975 is the period over which ref. 15 observed northern tree-ring density to diverge from temperature and to the period of Arctic dimming [12] , [14] ( Supplementary Fig. 1 ). Gridded results are obtained by averaging the mean trend in the residuals from each chronology within a grid box. Synthetic data experiments are used to compare the statistical power associated with the two approaches outlined in the foregoing paragraphs, referred to as BR1998 and SH2014, respectively. Each tree-ring density chronology i is represented as, The T i are temperature, each time series of which is realized as a red noise process having a power-law of 2 (that is, integrated white noise) and normalized to have zero mean and unit variance. The scaling of temperature is uniform over the entire domain, with a =1. L represents the process giving rise to dimming and is set to zero before 1955, a linear decrease from 1955–1975 to a value of minus one and again constant after 1975. Values of b i are specified to equal the actual light-limitation values nearest each tree-ring chronology, and are scaled such that the smallest value equals zero and the largest value equals 1.5. The n i are noise and are independently realized from a normal distribution having zero mean and unit variance. Values of c i are chosen to give, in expectation, the observed correlation between T and the tree-ring density chronologies for each site. Synthetic MXD records are generated following equation 1, after which the SH2014 and BR1998 methods are applied to each individual chronology. The Pearson’s correlation coefficient is then calculated between local light limitation, b , and both Briffa’s residual metric (divergence) and the 1955–1975 trend in residual density across the chronologies. This process is repeated 100,000 times to build up distributions for the correlation between light limitation and each residual metric. A distribution for the null hypothesis that the observed values of light limitation are unrelated to the residuals is obtained by randomly reordering the b values before computing correlation ( Supplementary Fig. 8 ). Although there are 263 individual chronologies included in our study, we use only 57 individual chronologies in computing each correlation, in accord with the 56 ESDOF estimated for the residual tree-ring density records. The 57 chronologies that are represented in each synthetic trial are randomly drawn from the pool of 263 without replacement in each Monte Carlo iteration. The statistical power of each test is the probability that it will identify a correlation between light limitation and each residual density metric given that the alternate hypothesis holds true. Using a significance level of P =0.05, the power of the SH2014 method is 0.80 and that of BR1998 is 0.48, indicating that the SH2014 methodology is much more likely to identify the influence of dimming on tree-ring density when such a relationship is truly present ( Supplementary Fig. 8 ). Both methods have a 5% probability of rejecting the null hypothesis when no relationship is present. This parameterization of the test gives results that are consistent with the results reported in the main manuscript. The maximum likelihood value for the SH2014 method agrees with the observed cross-correlation between trends in residual density and light limitation of 0.32 at the individual chronology level ( Supplementary Fig. 9 ). Note that the correlation is higher when averaging within grid boxes (see Fig. 3b ). The power of the test that we obtain does depend on the parameterizations of the synthetic test—including specification of the form and amplitude of variations in light availability, the distribution and variance of the noise and whether records are averaged—and other formulations also give consistent correlation. We have explored a large number of possible variations of this test, and in all plausible cases the SH2014 method is more likely to identify a relationship, should one in fact exist. The primary distinction between the two methods appears to be that the BR1998 method tends to amplify divergence most in those chronologies that have the weakest correlation with temperature. This leads to a fundamentally different representation of the spatial pattern of residual density changes. Indeed, the average correlation between the pattern of residuals estimated by the BR1998 and SH2014 methods for the synthetic data is small, at R =0.1. Application of these methods to the actual data also leads to patterns that are only weakly correlated ( R =0.27, Supplementary Fig. 10 ). This difference in how changes in residual tree-ring density are represented may help explain why the correspondence between light limitation and changes in tree-ring growth was not previously recognized. How to cite this article: Stine, A. R. & Huybers, P. Arctic tree rings as recorders of variations in light availability. Nat. Commun. 5:3836 doi: 10.1038/ncomms4836 (2014).